Causal mechanisms and balancing selection inferred from genetic associations with polycystic ovary syndrome Polycystic ovary syndrome (PCOS) is the most common reproductive disorder in women, yet there is little consensus regarding its aetiology. Here we perform a genome-wide association study of PCOS in up to 5,184 self-reported cases of White European ancestry and 82,759 controls, with follow-up in a further ∼ 2,000 clinically validated cases and ∼ 100,000 controls. We identify six signals for PCOS at genome-wide statistical significance ( P <5 × 10 −8 ), in/near genes ERBB4/HER4 , YAP1 , THADA , FSHB , RAD50 and KRR1. Variants in/near three of the four epidermal growth factor receptor genes ( ERBB2/HER2 , ERBB3/HER3 and ERBB4/HER4) are associated with PCOS at or near genome-wide significance. Mendelian randomization analyses indicate causal roles in PCOS aetiology for higher BMI ( P =2.5 × 10 −9 ), higher insulin resistance ( P =6 × 10 −4 ) and lower serum sex hormone binding globulin concentrations ( P =5 × 10 −4 ). Furthermore, genetic susceptibility to later menopause is associated with higher PCOS risk ( P =1.6 × 10 −8 ) and PCOS-susceptibility alleles are associated with higher serum anti-Müllerian hormone concentrations in girls ( P =8.9 × 10 −5 ). This large-scale study implicates an aetiological role of the epidermal growth factor receptors, infers causal mechanisms relevant to clinical management and prevention, and suggests balancing selection mechanisms involved in PCOS risk. Polycystic ovary syndrome (PCOS) is a common reproductive disorder in women that is defined by two out of three criteria: (1) menstrual irregularity (oligo-ovulation or anovulation), (2) hyperandrogenism (clinical or biochemical) and (3) polycystic ovarian morphology [1] , [2] . Phenotypic heterogeneity between cases has limited the ability to make definitive conclusions regarding its aetiology and pathophysiology. Obesity is associated with PCOS, but its causal role has yet to be determined [3] ; alternative explanations include reverse causality (that is, PCOS increases susceptibility to weight gain) and synergistic but independent roles for obesity and PCOS in infertility [4] . Hence, the role of lifestyle modification to prevent or reverse the reproductive abnormalities of PCOS is not well established [5] , [6] . Furthermore, although there is extensive evidence linking insulin resistance to PCOS, it is widely considered that the cellular and molecular mechanisms of insulin resistance in PCOS differ from those in other common insulin-resistant states such as obesity and diabetes [3] , [7] . Consequently, the role of insulin sensitisation therapy in PCOS remains limited to the prevention of cardiovascular disease and type 2 diabetes (T2D) [8] , [9] . Genetic studies could identify underlying genes and pathways, and thereby provide insights into the aetiology of PCOS. The results of candidate gene studies have been inconclusive, in large part due to underpowered studies, lack of replication and limited prior understanding of its pathogenesis [10] . Two, large genome-wide association studies (GWAS) for PCOS in overlapping Han Chinese populations identified in total 11 genomic loci [11] , [12] . Although these loci were enriched for candidate genes related to insulin signalling, steroid hormone regulation and T2D, and also for genes related to calcium signalling and endocytosis, the ability to make mechanistic interpretations from those findings was limited and only a few of these loci have been replicated in PCOS cases of European ancestry [13] , [14] , [15] , [16] , [17] . Furthermore, the striking paradox of a highly heritable yet common condition that impairs fertility has led to multiple theories for a balancing advantage of PCOS susceptibility [4] . Suggested mechanisms include enhanced fetal growth and development [18] or reproductive advantages, such as earlier pubertal maturation [19] or retarded ovarian ageing leading to a sustained reproductive lifespan [20] . Here we present a large-scale GWAS for PCOS in cases and controls of Caucasian European ancestry. As well as being the largest such study to date, we use dense imputation of genotypes to better implicate the probable genes underlying the association signals. As the GWAS is based on self-reported PCOS cases, we present follow-up in additional studies of clinically validated cases. We find six genetic loci associated with PCOS, highlighting aetiological roles for the epidermal growth factor receptors (EGFRs) and for the pituitary-derived gonadotrophins. Furthermore, using a genetic instrumental variable approach (i.e., Mendelian randomization) [21] , we infer causal roles in PCOS aetiology for higher body mass index (BMI), higher insulin resistance and lower serum sex hormone binding globulin (SHBG) concentrations. Finally, we find a robust association between menopause age-delaying alleles and higher risk of PCOS, suggesting a potential evolutionary advantage for PCOS genetic susceptibility. 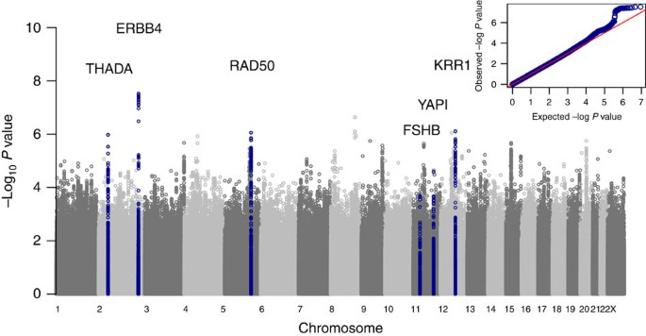Figure 1: Manhattan and QQ plots displaying PCOS genome-wide association results. Results shown are from discovery phase only. Genome-wide association signals for PCOS Six independent common signals reach genome-wide significance (logistic regression P <1 × 10 −8 ) for association with PCOS in the meta-analysis of discovery and follow-up studies ( Table 1 , Fig. 1 and Supplementary Fig. 1 ); four are novel signals and two represent refinements of previously reported signals at the YAP1 and THADA loci. 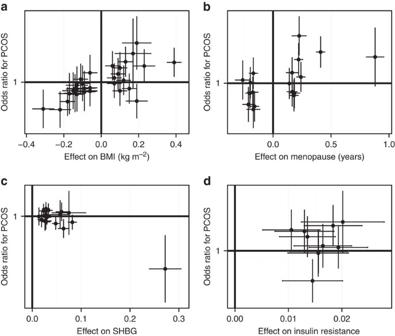Figure 2: Scatter plots of the associations between four significant intermediate traits. Panels show (a) BMI, (b) age at menopause, (c) SHBG and (d) insulin resistance, in each case showing the associations between the SNP and the trait of interest, and the odds ratio for PCOS for that SNP, with the attendant 95% confidence intervals. All signals show at least nominally significant ( P <0.05) directionally concordant associations in the follow-up studies of clinically validated PCOS cases, with no significant heterogeneity by PCOS case definition ( Supplementary Table 2 ). Table 1 Genetic variants associated with risk of PCOS. Full size table Figure 1: Manhattan and QQ plots displaying PCOS genome-wide association results. Results shown are from discovery phase only. Full size image Our strongest novel PCOS signal (rs1351592, odds ratio: 1.18 (1.13–1.23), P =1.2 × 10 −12 ) is intronic in ERBB4/HER4 , which encodes a member of the EGFR family. Notably, we find further sub-genome-wide significant signals in/near genes encoding two of the other three EGFR family members: rs7312770 ( P =2.1 × 10 −7 ) in/near ERBB3/HER3 is correlated ( r 2 =0.40) with the reported PCOS signal (rs705702) at 12q13.2 and rs7218361 ( P =9.6 × 10 −7 ) is a low-frequency variant ∼ 200 kb downstream of ERRB2/HER2 . Our second strongest novel signal (rs11031006, P =1.3 × 10 −9 ) lies near FSHB , which encodes the hormone-specific β-subunit of follicle stimulating hormone (FSH), a key promoter of ovarian follicle growth and oestrogen production. Interestingly, in deCODE samples, the PCOS-susceptibility allele at rs11031006 is also robustly associated with lower circulating FSH concentrations ( β =−0.089 s.d. per allele, P =9.2 × 10 −10 , n =15,586 women), higher luteinizing hormone (LH) concentrations ( β =0.115 s.d. per allele, P =3.6 × 10 −15 , n =17,469 women) and higher LH/FSH ratio ( β =0.272 s.d. per allele, P =5.94 × 10 −68 , n =14,310 women). This variant represents the strongest association signal for FSH, LH and LH/FSH ratio at this FSHB locus. Notably, a variant rs12294144 correlated with the PCOS risk allele is reportedly associated with later age at menopause [22] . Furthermore, FSH signalling was implicated in PCOS in the Han Chinese GWAS study through association with the FSH receptor gene FSHR [12] . However, that signal is only weakly associated with PCOS in our data ( Table 2 , rs2268361, P =1.6 × 10 −2 ). Table 2 PCOS associations in white Europeans for PCOS variants previously reported in Han Chinese. Full size table Our third novel signal (rs13164856, P =3.5 × 10 −9 ) is near RAD50 , which encodes a protein involved in DNA double-strand break repair. Fourth, rs1275468 ( P =1.9 × 10 −8 ) indicates a novel PCOS signal near KRR1 , which encodes a ribosome assembly factor. Previously reported PCOS loci Of the 11 PCOS signals reported in Han Chinese [11] , [12] , we observe directionally consistent associations for 10 variants, 6 of which are at least nominally associated ( P <0.05) in our discovery GWAS samples ( Table 2 ). Effect estimates are consistently smaller in our data, and in several instances the risk allele frequency is markedly different between these Han Chinese and white European populations. At three reported Han Chinese PCOS loci ( YAP1 , THADA and DENND1A ), we observe different lead signals in our white European samples ( Table 1 ). Our lead YAP1 signal, rs11225154 intronic to YAP1 , is highly correlated with the reported YAP1 signal ( r 2 =0.74 with rs1894116) and reaches genome-wide significance in our combined discovery and follow-up analysis ( P =7.6 × 10 −11 ). Our lead THADA signal, rs7563201 intronic to THADA , also reaches genome-wide significance ( P =3.3 × 10 −10 ) but is only weakly correlated with the reported THADA signal ( r 2 =0.08 with rs13429458). Our lead DENND1A signal (rs10760321) is also weakly correlated with the reported DENND1A signal ( r 2 =0.02 with rs2479106) but was not confirmed in our follow-up samples. These findings probably reflect differences in allelic structure between Chinese and European ancestry groups, as has been concluded by other investigators [15] , and limit the potential for conventional meta-analysis across these populations. Mendelian randomization analyses Our Mendelian randomization analyses indicate causal effects on PCOS aetiology for higher BMI (odds ratios: 1.90 per +1 s.d., 95% confidence interval: 1.55–2.34, P =2.5 × 10 −9 ), higher insulin resistance (1.11 per +1 s.d., 1.05–1.19, P =6 × 10 −4 ) and lower circulating SHBG concentrations (0.86 per +1 s.d., 0.78–0.93, P =5 × 10 −4 ) ( Table 3 ). Furthermore, the multiple allele score for menopausal age is positively associated with PCOS risk (1.60 per +1 s.d., 1.35–1.91, P =1.6 × 10 −8 ), indicating a common biological mechanism that promotes both PCOS susceptibility and later menopause. Our sensitivity analyses show apparent dose–response effects across individual single-nucleotide polymorphisms (SNPs) in each of these scores ( Fig. 2 ) and Funnel plots show no SNPs with outlier effects ( Supplementary Fig. 3 ). In contrast, we find no evidence for causal effects on PCOS for birth weight ( P =0.22) or age at menarche ( P =0.23). Table 3 Mendelian randomization analyses for PCOS risk. Full size table Figure 2: Scatter plots of the associations between four significant intermediate traits. Panels show ( a ) BMI, ( b ) age at menopause, ( c ) SHBG and ( d ) insulin resistance, in each case showing the associations between the SNP and the trait of interest, and the odds ratio for PCOS for that SNP, with the attendant 95% confidence intervals. Full size image Other biological mechanisms associated with PCOS By systematic testing of all GWAS SNPs across all known biological pathways using meta-analysis gene-set enrichment of variant associations (MAGENTA) software, we find one further pathway (ATP-binding cassette transporters) that is enriched for PCOS-associated variants. This pathway includes the genome-wide significant signal at the DNA repair gene RAD50 (rs13164856) and 37 other genes. The PCOS-susceptibility alleles at our six PCOS loci are also consistently associated with higher anti-Mullerian hormone (AMH) concentrations in girls (cumulative score: P =8.9 × 10 −5 ) ( Supplementary Fig. 3 ). However, none of these six genome-wide significant PCOS loci (nor any of the four suggestive loci) overlap with reported signals of positive selection and we can find no evidence of polygenic selection on the set of six loci considered together ( P =0.22) ( Supplementary Note ). Furthermore, these PCOS SNPs (or their proxies) are not associated with BMI (in aggregate: P =0.22). This large-scale genetic study reveals a number of insights into the aetiology and pathophysiology of PCOS. The findings from our Mendelian randomization analyses have perhaps most immediate relevance for treatment and prevention [21] , as these infer causal roles of greater BMI and insulin resistance. The role of interventions aimed at these targets in PCOS is debated. A recent US Endocrine Society Task Force found evidence that lifestyle modification reduces fasting blood glucose and insulin concentrations in women with PCOS but has uncertain effects on the key clinical features of PCOS, including reproductive outcomes [5] . The same conclusion was reached for the use of the insulin sensitizer Metformin in PCOS [5] , [23] . Conversely, a recent non-quantitative synthesis of dietary interventions positively concluded that weight-reducing diets have clinical benefits in PCOS [24] . The limitations of Mendelian randomization analyses are well-recognized; its major assumptions regarding lack of heterogeneity and pleiotropy are supported by the consistency of our findings across individual SNPs. Furthermore, the reported inverse association between the insulin resistance genetic score and BMI [25] might attenuate our observed positive univariate effects of these traits on PCOS risk. Other uncertainties remain, such as possible canalization and age-specific effects. Our findings should encourage the development and testing of more effective interventions to lower BMI and insulin resistance in women with PCOS. Our findings also infer a causal protective role of SHBG for PCOS, as has been reported for T2D [26] . SHBG regulates the bioavailability of testosterone. Therefore, genetic variants that lower circulating SHBG concentrations might directly modify the key hyperandrogenic phenotype of PCOS and also the related adverse metabolic profile [27] . Circulating SHBG concentrations rise markedly with the introduction of combined oral contraceptive pills, which are used by many women with PCOS for treatment of menstrual irregularity, acne and hirsutism [28] ; however, there are as yet no therapeutic agents that specifically target SHBG concentrations or activity. Despite the lack of any overlap between SNPs used in the SHBG and insulin resistance scores, it remains possible that these traits might lie on the same causal pathway, in which case joint interventions might have synergistic effects. Our novel genetic signals indicate a major role of the EGFRs in the pathogenesis of PCOS. There are four members of the EGFR family: EGFR, ERBB2, ERBB3 and ERBB4 (the last three are also known as the human epidermal receptors: HER-2, HER-3 and HER-4) [29] . These receptors form ligand-activated homo- or heterodimers with each other, which activates tyrosine kinase, and in cancer cells result in cell proliferation, blocking of apoptosis, activation of invasion and metastasis, and stimulation of neovascularization. EGFR signalling mediates LH-induced steroidogenesis, which in turn promotes late follicular maturation [30] , [31] . EGFRs are overexpressed in ovarian cancer [32] , [33] and repression of ERBB2/HER-2 determines the breast cancer response to the oestrogen receptor inhibitor tamoxifen [34] . Small molecules or monoclonal antibodies that block EGFR activation are effective cancer chemotherapy agents [29] . Variable reported associations between PCOS and risks of breast, endometrial and ovarian cancers are limited by small sample sizes and confounding due to related risk factors such as nulliparity, infertility and its treatment, anovulation and obesity [3] . Our findings provide a possible genetic link between PCOS and cancer risk, and also suggest potential ovary-targeted pharmaceutical interventions for treatment of PCOS. The novel PCOS locus at FSHB represents striking biological complementarity to the locus at the FSH receptor gene FSHR reported in Han Chinese [12] . However, the impact of that FSHR variant on FSH receptor activity is unclear and that locus shows only nominal association in our data, likely to be due to population differences in genetic architecture. Non-synonymous variants in FSHR that confer lower FSH receptor activity are inconsistently associated with PCOS [35] . We show that the PCOS-susceptibility allele at FSHB is robustly associated with a higher LH/FSH ratio, which is the hallmark biochemical PCOS trait that promotes ovarian androgen production and arrests follicular growth [36] . Although the high LH/FSH ratio observed in PCOS might be exacerbated by central feedback effects of peripheral hyperandrogenemia [37] , our findings establish a co-primary neuroendocrine pathogenesis of PCOS. Our findings inform the long-standing debate regarding the evolutionary paradox of PCOS as a common yet highly heritable disorder characterized by infertility. We cannot find evidence for recent, strong positive selection of PCOS-susceptibility alleles; however, available tests may be insensitive to detect signals that affect complex traits [38] , [39] . The robust association between menopause age-raising alleles and PCOS susceptibility implicates a common mechanism that retards ovarian ageing. GWAS studies for age at menopause has highlighted a key role for DNA repair pathways [22] , [40] and their putative relevance to PCOS is supported by the novel PCOS locus near to RAD50 , a gene that is involved in DNA double-strand break repair and is mutated in the Nijmegen breakage syndrome-like disorder. Anovulation in women with PCOS is characterized by arrested follicle growth at the early antral stage, when AMH secretion from follicular granulosa cells is highest. Higher AMH concentrations consequently inhibit the recruitment of further primordial follicles, possibly representing more efficient use of the primordial ovarian pool [20] . This mechanism could possibly explain the consistent association we find between PCOS-susceptibility alleles and higher serum AMH concentrations, and might be a further mechanism towards slower ovarian ageing. Alternatively, higher AMH concentrations could indicate a larger ovarian primordial follicle pool size [4] . Such evolutionary debates are not just interesting arguments, but may be eventually informative to clinical practice. The anticipated persistence of reproductive lifespan may inform the use of artificial reproductive therapies or long-term lifestyle intervention strategies in women with PCOS. Progress in identifying PCOS-susceptibility variants has been slow compared with other complex diseases, in part due to the relatively small collections of cases [10] . We demonstrate here, as previously reported for other traits [41] , that online self-reports of disease status is a highly efficient study design to identify large numbers of disease cases, providing sufficient power to identify robust genetic signals for PCOS. This is evident by our confirmation of previously identified PCOS signals in Han Chinese, by the highly consistent validation of our novel loci in cases defined by stringent clinical criteria and by the lack of heterogeneity in variant effect sizes between these case groups. That said, it remains important to confirm any findings of self-reported case studies in clinically validated cases. The range of biological mechanisms that we can currently test by Mendelian randomization is limited by available GWAS findings. In particular, future analyses are needed to investigate the roles of androgen production and activity once robust genetic markers for those traits are identified. Indeed, we anticipate that future genetic instruments will allow wider and deeper testing of causal biological pathways. Although such analyses cannot infer possible developmental stage-specific effects of these pathways, the findings should encourage experimental studies that target these pathways, both to confirm the causal inferences and also to inform effective intervention and preventive strategies. In conclusion, this genetic study reveals new biological and evolutionary insights into the pathogenesis of PCOS, including a major role of EGFRs, a co-primary neuroendocrine pathogenesis and genetic mechanisms towards slower ovarian ageing. Furthermore, the causal inferences from our Mendelian randomization analyses should support future efforts to develop and test effective interventions, to reduce body weight and insulin resistance in the treatment and prevention of PCOS. Discovery phase Genome-wide SNP data were available on 5,184 women of White European ancestry with self-reported PCOS and 82,759 controls from the 23andMe study (see Supplementary Table 1 and Supplementary Note for details of the 23andMe study). Imputation was performed against the 1000 Genomes reference (March 2012 v3 release), yielding ∼ 9 M variants that passed imputation and minor allele frequency criteria. A logistic regression model adjusting for age- and study-specific principal components was performed assuming an additive allelic model including covariates for age and the top five principal components to account for residual population structure. Test statistics were further adjusted for the observed λ -value 1.041. 23andMe participants provided informed consent to take part in this research under a protocol approved by Ethical and Independent Review Services, an accredited institutional review board. Follow-up studies From our discovery GWAS phase results, we selected for follow-up in additional studies: (a) all signals that showed at least suggestive associations ( P <1 × 10 −6 ) with PCOS ( N =5 signals, where a signal is defined by the most significant SNP within a 1-Mb window; Table 1 ); (b) all possible signals for PCOS ( P <1 × 10 −5 ) located within 500 kb of signals previously reported in Han Chinese ( N =3 signals; in/near YAP1 , THADA and DENND1A ); and (c) possible signals for PCOS near to biological candidate genes ( N =2 signals; in/near ERBB2/HER2 and FSHB ). Follow-up was performed in three independent studies of clinically validated PCOS cases and control women: deCODE, Rotterdam and Boston (see Supplementary Table 1 and Supplementary Note for details and parameters of follow-up studies). Separate follow-up analyses were performed using PCOS case definitions either by Rotterdam 2003 criteria [1] (1,875 cases from Rotterdam and deCODE) or by NIH criteria [2] (861 cases from Boston and deCODE). Final association test statistics were produced from a combined meta-analysis of 7,229 cases and 181,645 controls across non-overlapping discovery and follow-up (2,045 cases and 98,886 controls) samples; as the two PCOS groups in deCODE include overlapping cases, only deCODE cases defined by NIH criteria were included in this combined meta-analysis. The follow-up studies were approved by local research ethics committees and all participants provided informed consent. Mendelian randomization analyses Mendelian randomization is an analytical method to infer the unconfounded causal relationship between an exposure trait and an outcome, using genetic variants that are associated with the exposure trait and do not influence the outcome by other unrelated biological pathways (‘pleitropy’) [21] . In both the 23andMe and Rotterdam studies, we approximated weighted multiple allele scores (single variables summarizing multiple genetic variants associated with a risk factor, as described by Dastani et al . [42] ), to represent genetic instrumental variables for 15 traits (birth weight, BMI, height, age at menarche, age at menopause, dehydroepiandrosterone sulphate, SHBG, total cholesterol, high-density lipoprotein cholesterol, low-protein lipoprotein cholesterol, triglycerides, systolic and diastolic blood pressure, insulin resistance and insulin secretion) based on reported GWAS signals for those traits. Each score was calibrated to a 1-s.d. change in the exposure trait, using the published effect estimates of individual alleles on those traits in the replication stages of those GWAS reports ( Supplementary Table 3 ). To account for the multiple traits tested, we set a corrected P -value threshold (0.05/15=0.0033) to indicate statistically significant associations. To test for pleiotropy, which can invalidate inferences from Mendelian randomization, we performed sensitivity analyses to examine the consistency in causal estimates derived from individual SNPs. Serum AMH concentrations The cumulative influence of PCOS-associated variants on childhood serum AMH concentrations, a marker of ovarian primordial follicle pool size [4] , was estimated by analysis of data in 1,455 girls (aged 15 years) from the ALSPAC study [43] . Serum AMH concentrations (ng ml −1 ) were natural log transformed before analysis in an additive linear regression framework. Tests for positive selection Allelic variants that increase the reproductive fitness of their carriers should become more prevalent in the population. The resulting genomic characteristics of strong recent positive selection include low haplotype diversity, high linkage disequilibrium and marked shifts in allele frequency between populations. However, there is often poor consistency between signals identified from available tests [38] , [39] . We therefore looked for evidence of selection at the ten PCOS loci in Table 1 , using various strategies. We investigated whether any of the lead SNPs overlapped with signals of positive selection identified in 1000 Genomes data using the composite of multiple signals test [44] . None of the lead PCOS SNPs lies in any of the 424 non-overlapping regions with evidence of positive selection, a total of 19 Mb of sequence ( http://www.broadinstitute.org/mpg/cmsviewer/download/cms_localized_regions_062712.txt ). Three of the ten signals lie within 1 Mb of one of these regions (a total of 726 Mb of sequence), which is not more than expected by chance ( P =0.56 assuming an accessible genome length of 2.6 Gb). We tested whether the lead PCOS SNPs are more differentiated across populations compared to with randomly chosen loci, using the test described by Berg and Coop [45] , and Omni chip data from phase 1 of the 1000 Genomes Project [46] as a reference panel ( ftp://ftp-trace.ncbi.nih.gov/1000genomes/ftp/phase1/analysis_results/supporting/omni_haplotypes/ ). As only two of the ten PCOS SNPs were genotyped by the Omni chip, we added the remaining eight SNPs from the sequence data. Using 10,000 bootstrap replicates of SNP frequency matched in 20 bins, we find no evidence of polygenic selection in European ( P =0.38), Asian ( P =0.37), or combined European and Asian ( P =0.42) populations. We also tested PCOS susceptibility variants with minor allele frequency >0.2 using the integrated haplotype score [38] , which measures the difference in haplotype homozygosity associated with the ancestral and derived alleles, and the derived intra-allelic nucleotide diversity test [38] , which measures the differences in nucleotide diversity associated with the ancestral and derived alleles. We find no significant test statistics ( P <0.01). Pathway analyses MAGENTA ( https://www.broadinstitute.org/mpg/magenta/ ) was used to test for enrichment of genome-wide SNP associations with PCOS in pre-defined biological pathways (Gene Ontology, PANTHER, KEGG and Ingenuity) using the full discovery data set. MAGENTA implements a gene-set enrichment analysis-based approach, where each gene throughout the genome is mapped to a single index SNP with the lowest P -value within a 110-kb upstream and 40-kb downstream window. This P -value, representing a gene score, is then corrected for confounding factors such as gene size, SNP density and linkage disequilibrium (LD)-related properties in a regression model. Genes within the human leukocyte antigen region were excluded from analysis, owing to difficulties in accounting for gene density and LD patterns. Each gene is then ranked by its adjusted gene score. At a given significance threshold (95th or 75th percentiles of all gene scores), the observed number of gene scores in a given pathway, with a ranked score above the specified threshold percentile, is calculated. This observed statistic is then compared with 1,000,000 randomly permuted pathways of identical size. This generates an empirical gene-set enrichment analysis P -value for each pathway. In total, 2,529 pathways were tested for enrichment of multiple modest associations with PCOS. Significant pathways are indicated by a false discovery rate <0.05 in either model (95th or 75th percentiles). How to cite this article: Day, F. R. et al . Causal mechanisms and balancing selection inferred from genetic associations with polycystic ovary syndrome. Nat. Commun. 6:8464 doi: 10.1038/ncomms9464 (2015).